Hierarchical micro/nanostructured silver hollow fiber boosts electroreduction of carbon dioxide Efficient conversion of CO 2 to commodity chemicals by sustainable way is of great significance for achieving carbon neutrality. Although considerable progress has been made in CO 2 utilization, highly efficient CO 2 conversion with high space velocity under mild conditions remains a challenge. Here, we report a hierarchical micro/nanostructured silver hollow fiber electrode that reduces CO 2 to CO with a faradaic efficiency of 93% and a current density of 1.26 A · cm −2 at a potential of −0.83 V vs . RHE. Exceeding 50% conversions of as high as 31,000 mL · g cat −1 · h −1 CO 2 are achieved at ambient temperature and pressure. Electrochemical results and time-resolved operando Raman spectra demonstrate that enhanced three-phase interface reactions and oriented mass transfers synergistically boost CO production. Large-scale CO 2 utilization, abating carbon emissions while producing commodity chemicals, is a promising strategy for achieving carbon neutrality [1] , [2] , [3] . Thermocatalytic routes such as CO 2 hydrogenation to methanol or other compounds exhibit industrial potential but suffering from the dilemmas of hydrogen sources and severe reaction conditions [4] , [5] , [6] . Recently, electrocatalytic CO 2 conversion has emerged as a remarkable technology that benefits from the desirable coupling of renewable electricity transition and CO 2 utilization [7] , [8] , [9] , [10] . However, the efficiency of CO 2 electroreduction is much inferior to thermocatalytic CO 2 conversion processes due to the limited CO 2 solubility in electrolyte solutions and divergent kinetics [9] , [11] . One tactic for addressing these issues is adopting gas-diffusion electrodes that consist of highly active catalysts decorated with superhydrophobic polytetrafluoroethylene and conductive carbon layers [12] , [13] , [14] , [15] . Regarding such gas-diffusion electrodes, these multiple components are assembled via subtle procedures to build complicated configurations, which could hinder their practical scale-up. 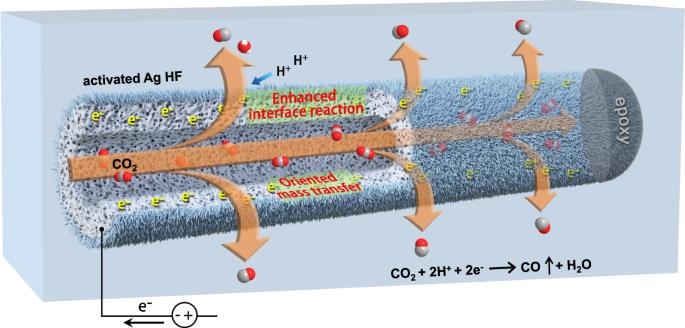Fig. 1: Function outline of hollow-fiber silver electrode. Schematic illustration of hierarchical micro/nanostructured silver hollow fiber for boosting CO2electroreduction to CO. Although large current densities and high faradaic efficiencies of various products have been realized over these gas-diffusion electrodes [12] , [16] , their CO 2 conversion rates especially at high flow rates are still lower than 20% (Supplementary Table 1 ). Furthermore, three-dimensional hollow fiber electrodes with a compact structure exhibit promising potentials in efficient and high-rate CO 2 electroreduction by virtue of improved mass transport [17] , [18] , [19] , [20] , [21] . To date, the hollow fiber electrodes still deliver too limited current densities (≤200 mA ∙ cm −2 ) to afford an economically viable CO 2 electrochemical conversion [19] , [20] . Herein, we report a hollow fiber electrode with hierarchical micro/nanostructures composed of only metallic silver (Ag) for electroreducing CO 2 to CO. Such a porous hollow-fiber Ag electrode acting as a CO 2 disperser can not only enhance three-phase interface reactions but also guide mass transfers during electrolysis (Fig. 1 ). As a result, CO 2 conversions exceed 50% at a high space velocity of 31,000 mL ∙ g cat −1 ∙ h −1 corresponding to a flow rate of 60 mL ∙ min −1 under ambient conditions, maintaining stable large current densities (~1.26 A ∙ cm −2 ) and high CO faradaic efficiencies (~93%) in a continuous test for a long lifespan, and this represents an encouraging headway in sustainable CO 2 utilization. Fig. 1: Function outline of hollow-fiber silver electrode. Schematic illustration of hierarchical micro/nanostructured silver hollow fiber for boosting CO 2 electroreduction to CO. Full size image Structure and composition The silver hollow fiber (Ag HF) was first fabricated by a combined phase-inversion/sintering process from commercial Ag powder (Supplementary Fig. 1 ), followed by electrochemical redox activation treatments to obtain an activated Ag HF (Supplementary Figs. 2 – 4 ). The fused silver particles from the outer surface of Ag HF rather than spherical ones in pristine Ag powder (Supplementary Figs. 5 , 6 ) implied that a well-integrated substrate was formed by sintering during Ag HF fabrication. The surfaces of the slender Ag HF tubes exhibited metallic luster (Fig. 2a ), and their scanning electron microscopy (SEM) images showed abundant micrometer-sized pores on the outer/inner surfaces and interconnected pores inside the wall of Ag HF (Fig. 2b, c and Supplementary Figs. 5b , 7a ). By the electrochemical activation treatments to reconstruct the outer surface of Ag HF, partly ordered nanorods gathered at the outer region, configuring hierarchical micro/nanostructures in activated Ag HF (Fig. 2d, e and Supplementary Fig. 7b ). The effective porosities of Ag HF and activated Ag HF, as determined by gas permeation tests, were 38% and 32%, respectively (Supplementary Fig. 8 and Fig. 2f ). Both X-ray diffraction (XRD) (Fig. 2g ) and X-ray photoelectron spectroscopy (XPS) (Fig. 2h ) verified that the bulk and surface compositions of Ag HF and activated Ag HF were identical with metallic silver (Supplementary Figs. 9 , 10 ). Fig. 2: Structural and compositional characterization. a Optical image of the as-fabricated Ag HF tubes. SEM images of b , d , cross sections and c , e , outer surfaces of b , c , Ag HF and d , e , activated Ag HF. Scale bars in b , c , d and e are 50 µm, 5 µm, 10 µm and 500 nm, respectively. f Gas permeances of activated Ag HF. GPU denotes gas permeation unit. Inset: the permeances (at 1.0 bar) are proportional to the inverse square root of gas molecular weight. g XRD patterns, and h , XPS spectra of Ag HF and activated Ag HF. Full size image Electrocatalytic performance The Ag HF array comprising ten tubes was used as the working electrode (Supplementary Fig. 11 ) and subjected to the potentiostatic electrolysis of CO 2 after the electrochemical activation treatments. Over a single tube of the activated Ag HF electrode, CO 2 molecules were highly dispersed via penetrating through the porous wall of activated Ag HF, and CO was produced at the gas-liquid-solid three-phase interface sites (Fig. 1 ). The CO partial current density ( j CO ), i.e., the total current density × CO faradaic efficiency, showed superior in the relatively concentrated solutions with the best performance in 1.5 M KHCO 3 (Supplementary Fig. 12 ). On basis of the intrinsic structure characteristics of activated Ag HF, the CO 2 flow rate was fixed at 60 mL ∙ min −1 during CO 2 electroreduction to obtain the optimal electrocatalytic performance (Supplementary Fig. 13 ). As shown in Fig. 3a , only CO and H 2 were detected over the activated Ag HF electrode (Supplementary Fig. 14 ) with their faradaic efficiency sum almost equaling 100% in the potential range of −0.35 to −0.89 V. The H 2 faradaic efficiency was always less than 3% up till −0.72 V while the total current density kept growing rapidly. At −0.83 V, the CO faradaic efficiency was 93% with the total current density of 1.26 A ∙ cm −2 . Then, the CO faradaic efficiency dropped down to 83% at −0.89 V, although the total current density increased to 1.69 A ∙ cm −2 , implying a rising hydrogen evolution reaction (HER) at more negative potentials. Further evaluation of the durability of the activated Ag HF electrode was performed in a continuous CO 2 electrolysis test operated at −0.83 V. The CO faradaic efficiency remained between 93 and 92% and the total current density fluctuated between 1.26 and 1.24 A ∙ cm −2 , manifesting no declining sign for 170 h (Fig. 3b ). The postreaction XRD (Supplementary Fig. 9 ) and XPS (Supplementary Fig. 10 ) revealed the unchanged compositions of activated Ag HF after the electrolysis, and the corresponding structural features were also highly similar to those before the electrolysis (Supplementary Fig. 8 ), which were responsible for the stable CO 2 electroreduction performance. Fig. 3: Performance of activated Ag HF. a CO and H 2 faradaic efficiencies, and total current densities in the potential range of −0.35 to −0.89 V. Error bars in a were obtained from the average of six individual tests. b Long-term performance at −0.83 V. c CO 2 conversion rates with a space velocity of 31,000 mL · g cat −1 · h −1 at different current densities, and their overall comparison with other electrocatalytic and thermocatalytic CO 2 conversions. All comparison data points in c are from the references summarized in Supplementary Table S1 , and the key data points are referred to the corresponding Supplementary references Srx, where x represents the reference number in Supplementary Information . CO 2 -saturated 1.5 M KHCO 3 as the electrolyte solution, and the CO 2 flow rate of 60 mL · min −1 . Full size image CO 2 conversion rate is an important common criterion for both thermocatalytic and electrocatalytic processes, and their overall comparisons are displayed in Fig. 3c . In the current density range from 2 to 400 mA ∙ cm −2 , the CO 2 conversion rates of activated Ag HF were comparable to those over other prominent catalysts reported in electrocatalysis. Note that the CO 2 conversion rates further increased rapidly with negative-shifting potentials (Supplementary Fig. 15 ) and increasing current densities, which approached the theoretical predictions, far outperforming the previously reported electrocatalysts (Fig. 3c and Supplementary Table 1 ). At −0.83 V, the CO 2 conversion rate of activated Ag HF was 54% with sustained performance during the long-term test (Fig. 3b ). Furthermore, the thermocatalytic catalysts run at high temperature (170–360 °C) and pressure (1–5 MPa) delivered relatively low CO 2 conversion rates (less than 22%) at high space velocities (≥18,000 mL ∙ g cat −1 ∙ h −1 ) (Fig. 3c and Supplementary Table 1 ). In contrast, the CO 2 conversion rates over the activated Ag HF electrode at CO 2 space velocity of 31,000 mL ∙ g cat −1 ∙ h −1 exceeded 28% just from −0.72 V and 54% from −0.83 V under ambient conditions, even higher than those over low-space-velocity-run catalysts of CO 2 hydrogenation (Supplementary Fig. 15 and Supplementary Table 1 ). Previous studies [22] , [23] , [24] , [25] reported Ag electrocatalysts possessing the capability to selectively reduce CO 2 to CO, but their current densities of long-term tests remained below 200 mA∙cm −2 (Supplementary Table 1 ), far from the ≥400 mA ∙ cm −2 regime for industrial applications [26] , [27] . In sharp contrast, our activated Ag HF electrode manifested the sustained large current density (~1.26 A ∙ cm −2 ) with high CO faradaic efficiency (~93%), implying a striking promotion in the intrinsic activity of Ag. Electrochemical characterization The electrochemically active surface areas (ECSAs) of activated Ag HF, Ag HF, activated Ag foil and Ag foil were determined by measuring their double-layer capacitance ( C dl ) values via their cyclic voltammetry curves (Supplementary Fig. 16 ). Although the ECSA of activated Ag HF was only nearly 3 times that of activated Ag foil (Fig. 4a ), the j CO of activated Ag HF with the lower overpotential was almost two orders of magnitude larger than that of activated Ag foil (Fig. 4b and Supplementary Fig. 17 ). This implied that the high ECSA only played a secondary role in efficiently producing CO over activated Ag HF. Fig. 4: Electrochemical characterization. a Plot of Δj (the difference of cathodic and anodic current densities, j c – j a ) against the scan rates from cyclic voltammetry curves (Supplementary Fig. 16 ), b CO partial current density comparison, and error bars were obtained from the average of six individual tests. c EIS Nyquist plots of activated Ag HF, Ag HF, activated Ag foil and Ag foil. The inset in c shows the equivalent circuit. Full size image Furthermore, the electrochemical impedance spectroscopy (EIS) measurements were performed to study the electron transfer behaviors of the activated Ag HF, Ag HF, activated Ag foil and Ag foil electrodes, and their impedance spectra in the complex plane (Nyquist plot) are presented in Fig. 4c . The activated Ag HF electrode exhibited the smallest R ct (0.2 Ω ∙ cm 2 ) compared with those of Ag HF (2.5 Ω ∙ cm 2 ), activated Ag foil (7.8 Ω ∙ cm 2 ) and Ag foil (25.4 Ω ∙ cm 2 ), indicating the most favorable CO 2 reduction kinetics over activated Ag HF. CO 2 dispersion effects In comparison with other counterparts, activated Ag HF was distinguished in that it possessed the unique CO 2 diffusion manner acting as a CO 2 disperser. That is the restrained environment of activated Ag HF offered a scenario that CO 2 were compulsively interacted with active sites when penetrating through the porous wall (Fig. 5a ), resulting in enhanced three-phase interface reactions and optimized kinetics to produce CO efficiently. Obviously, such CO 2 dispersion effects of activated Ag HF vanished just switching to non-CO 2 -disperser mode (Fig. 5a, b ). The comparison of CO partial current densities over the activated Ag HF electrode with the CO 2 -disperser and non-CO 2 -disperser modes is shown in Fig. 5b . As the potential negatively shifted from −0.35 to −0.94 V, the j CO of activated Ag HF using the CO 2 -disperser mode increased quickly and reached the maximum value of 1402 mA ∙ cm −2 at −0.89 V, then slightly decreased to 1268 mA ∙ cm −2 at −0.94 V. In sharp contrast, activated Ag HF using the non-CO 2 -disperser mode always delivered rather low j CO values and showed a maximum value of only 33 mA ∙ cm −2 at −1.07 V. These results indicated that the CO 2 -disperser mode was uniquely superior to the non-CO 2 -disperser mode. Fig. 5: CO 2 dispersion effect studies. a Schematic illustrations showing the processes of CO 2 electroreduction over activated Ag HF with the CO 2 -disperser mode and the non-CO 2 -disperser mode, respectively, and b , their CO partial current densities. Error bars in b were obtained from the average of six individual tests. c Tafel slopes of activated Ag foil and activated Ag HF with different dispersion modes. Full size image It is generally known that large current densities in water-based electrolytes will lead to the high local pH near the electrode surface, which inhibits the HER and increases CO 2 reduction due to the proton depletion [28] , [29] , [30] . Besides such CO 2 reduction promotion from local pH variation, our activated Ag HF electrode could deliver large and stable current density lying in the enhanced three-phase interface reactions and mass transfers. That is the high-flow-rate CO 2 rushing out from the porous hollow fiber wall to react on the abundant active Ag nanorods at the outer region, thereby maintaining extremely high local CO 2 concentration at three-phase interface sites for significant CO 2 electroreduction rather than HER [31] , [32] . Consequently, such a hollow fiber dispersion design maximizes the efficiency of the three-phase reaction interfaces, showing a promising potential compared with the conventional membrane electrode assembly. Furthermore, a comparison of the kinetic data extracted from the Tafel plots, namely, the overpotential ( η ) versus log( j CO ), was made for activated Ag foil and activated Ag HF with the non-CO 2 -disperser and CO 2 -disperser modes, as shown in Fig. 5c . In the low overpotential regime (i.e., Tafel linearity) of −140 to −290 mV, a Tafel slope of 113 mV ∙ dec −1 was obtained for activated Ag foil, close to the value of 118 mV ∙ dec −1 expected for a rate-determining single-electron transfer at the electrode surface [33] . This result indicated that the initial one-electron transfer for CO 2 activation over activated Ag foil to form an adsorbed *COO − intermediate (Supplementary Fig. 18 ) was the rate-determining step, in consistence with previous reports [33] , [34] . Furthermore, a dramatically increased Tafel slope for activated Ag foil was observed at relatively high overpotentials, implying that CO 2 electroreduction likely reached a mass transfer limitation [34] , [35] . In contrast, activated Ag HF with the CO 2 -disperser mode showed the smallest Tafel slope (63 mV ∙ dec −1 ), close to the theoretical value of 59 mV ∙ dec −1 [35] , [36] , suggesting a fast initial one-electron transfer step to form *COO − and a subsequent slower chemical reaction as the rate-determining step (Supplementary Fig. 18 ). The Tafel slope of activated Ag HF with the CO 2 -disperser mode at high overpotential regime was also much smaller than that of activated Ag foil, implying the favorable mass transfer. Interestingly, the Tafel slope for activated Ag HF with the non-CO 2 -disperser was 108 mV ∙ dec −1 , which was close to the value of 113 mV ∙ dec −1 for activated Ag foil. This result indicated that both had the same rate-determining step, namely, the initial one-electron transfer, which also confirmed the superiority of the CO 2 -disperser mode for CO 2 reduction. In addition, the high-overpotential Tafel slope for activated Ag HF with the non-CO 2 -disperser mode was closer to that for activated Ag foil. These results indicated that the improved initial one-electron transfer and mass transfer jointly enhanced the intrinsic CO 2 reduction activity of activated Ag HF with the CO 2 -disperser mode, resulting in high selectivity and activity for the electrocatalytic reduction of CO 2 to CO. Mechanistic studies Isotope-labelling experiments were conducted using C 18 O 2 and D 2 O as feedstocks to reveal the mass migrations involved in CO 2 electroreduction over activated Ag HF. The results in Fig. 6a and Supplementary Fig. 19 suggested that CO production was derived from the CO 2 dissociation to form one O atom, which coupled with two protons (H + ) to generate H 2 O (Fig. 5a ), while anodic water oxidation released and supplied protons to participate in cathodic CO 2 reduction. This indicated that the product CO originated from the reduction of CO 2 and the anodic reaction maintained the proton and charge balances of the overall CO 2 electroreduction reaction. Fig. 6: Isotopic trace and time-resolved operando Raman results. a Mass spectrometric detections of the cathodic products over activated Ag HF using unlabeled feedstocks (upper) and isotopically labeled C 18 O 2 and D 2 O feedstocks (lower), respectively. b , c Time-resolved operando Raman spectra showing the formation, evolution and dissipation of intermediates over activated Ag HF. d Comparison of the normalized *COO − peak intensities of activated Ag HF and activated Ag foil during the power-on and power-off stages. Full size image Time-resolved operando Raman spectroscopy was resorted to further reveal the formation and evolution of key intermediates during CO 2 electroreduction. The typical operando Raman spectra of both activated Ag HF and activated Ag foil (Supplementary Fig. 20 ) showed two Raman bands at 532 and 390–410 cm −1 , corresponding to adsorbed *COO − and *COOH intermediates, respectively [37] , [38] , besides bicarbonate ion related peaks above 1000 cm −1 [39] , [40] , [41] . The chronological appearances of *COO − and *COOH (Fig. 6b and Supplementary Fig. 21c ) implied the step-by-step reduction of CO 2 , i.e., the initial step to form *COO − and the second step to form *COOH, in agreement with the proposed mechanism (Supplementary Fig. 18 ). After power-on for 720 ms ( t1 ), *COO − Raman peak over activated Ag HF appeared, and then its intensity increased quickly and reached the maximum at 2720 ms ( t2 ) (Fig. 6b and d). Regarding activated Ag foil, the *COO − peak appeared at 660 ms ( t1’ ), and the peak intensity reached a maximum at 3080 ms ( t2’ ) (Supplementary Fig. 21c and Fig. 6d ). Compared to activated Ag foil, more *COO − intermediates were formed and adsorbed over activated Ag HF in a shorter time (Fig. 6d and Supplementary Figs. 21a, c ), implying the superior capability of CO 2 activation over activated Ag HF, which probably profited from the reduced CO 2 diffusion distance in the CO 2 -disperser mode. Subsequently, we investigated the variation of adsorbed *COO − over activated Ag HF and activated Ag foil during the power-off stages (Fig. 6c and Supplementary Fig. 21d ). As soon as the power was off, the 532 cm −1 ν *COO - redshifted abruptly for both electrodes due to the Stark effect [41] , [42] , [43] , [44] , indicating the distinct impact of electric field on the adsorption of intermediates (Supplementary Fig. 22 ). The *COO − peak vanished over activated Ag HF after power-off for 1050 s ( t3 ) (Fig. 6c, d ), whereas over activated Ag foil after power-off for 1400 s ( t3’ ) (Supplementary Fig. 21d and Fig. 6d ). Moreover, the dissipation time of *COO − over activated Ag HF with non-CO 2 -disperser mode was 1380 s ( t3” ) (Supplementary Fig. 23 ), which was close to that (1400 s, t3’ ) over activated Ag foil. The faster dissipation of adsorbed *COO − benefited from the one-way CO 2 flow manner of activated Ag HF with the CO 2 -disperser mode (Fig. 6d ). While direct Raman observations on the formation and desorption of *CO species were not available at present, to be explored in further study. Consequently, these Raman results suggested that the oriented mass transfers induced by the CO 2 -disperser mode of activated Ag HF could not only favor the diffusion of CO 2 to active sites but also facilitate the desorption of adsorbed species from the electrode surface, resulting in the improved overall kinetics of CO 2 reduction. Our results demonstrate that the electrocatalytic performance of CO 2 reduction could be greatly improved by adopting the micro/nanostructured hollow fiber configuration of silver, which provides new opportunities for heightening three-phase interface reactions and mass transfer kinetics simultaneously. In addition, the single composition and tough framework with simple fabrication procedures enable activated Ag HF to become an ideal industrial electrode with excellent durability. This work represents an encouraging headway in CO 2 electroreduction that may lead to scalable applications. See the Supplementary Information for detailed description of the methods employed in this study. Chemicals and materials Ag powder (99.9%, 50 nm) was purchased from Ningbo Jinlei Nano Materials Co., Ltd. Ag foil (99.9%, 1 mm thick) was purchased from Shanghai Macklin Biochemical Technology Co., Ltd. Polyetherimide (PEI) was purchased from Saudi Basic Industries Corporation (SABIC). N-Methyl-2-pyrrolidone (NMP) and potassium bicarbonate (KHCO 3 ) were purchased from Sinopharm Chemical Reagent Co., Ltd. Nafion 117 proton exchange membranes (PEM) with an average thickness of 183 µm were purchased from DuPont. 3-Trimethylsilyl-1-propane sulfonic acid sodium salt (DSS) was purchased from Sigma-Aldrich. Isotope-labeled C 18 O 2 (purity: 97 at.%) was purchased from Sigma-Aldrich. Deuterium oxide (D 2 O) was purchased from Sigma-Aldrich. All chemicals were used as received without further purification. Electrolyte solutions were prepared using 18.2 MΩ H 2 O (ultrapure water, from Master-S30UVF water purification system). Catalyst preparation Ag HF was first fabricated by a combined phase-inversion/sintering process, and then was treated by electrochemical redox activation to obtain activated Ag HF. More details can be found in Supplementary Preparations section as well as Supplementary Figs. 1 and 2 . Physical characterization The cross-section and surface morphologies were observed by scanning electron microscopy (SEM) with a SUPRRATM 55 microscope using an accelerating voltage of 5.0 kV. Transmission electron microscopy (TEM) investigations were conducted with a JEM-ARM300F microscope operated at 300 kV. X-ray diffraction (XRD) measurements were performed on a Rigaku Ultima 4 X-ray diffractometer using a Cu Kα radiation source (λ = 1.54056 Ǻ) at 40 kV and 40 mA. X-ray photoelectron spectroscopy (XPS) was conducted using a Quantum 2000 Scanning ESCA Microprobe instrument with a monochromatic Al Kα source (1486.6 eV). The binding energies in all XPS spectra were calibrated according to the C 1 s peak (284.8 eV). Electrochemical characterization Electrochemical characterization was performed on a Biologic VMP3 potentiostat in a gas-tight two-compartment electrolysis cell equipped with a KCl-saturated Ag/AgCl reference electrode and a platinum mesh (3 cm × 3 cm) counter electrode. The electrochemically active surface area (ECSA) of the electrode was evaluated by the double-layer capacitance ( C dl ). The C dl was determined by performing cyclic voltammetry (CV) in the potential range of 0.4 to 0.5 V ( vs . RHE) at different scan rates in CO 2 -saturated 1.5 M KHCO 3 . The electrochemical impedance spectroscopy (EIS) measurements were performed in CO 2 -saturated 1.5 M KHCO 3 at −0.83 V ( vs . RHE), and the frequency limits were typically set in the range of 0.1 Hz to 100 kHz with a voltage amplitude of 10 mV. Prior to the experiments, the electrolysis cell was vacuumized and then purged with CO 2 for 30 min, after which CO 2 was continuously delivered into the cathodic compartment at a constant rate of 10 mL · min −1 . All the applied potentials were recorded against the KCl-saturated Ag/AgCl reference electrode and then converted to those versus the reversible hydrogen electrode (RHE) with iR compensation by the following equation: \(E\left({vs}.{RHE}\right)=E\left({vs}. 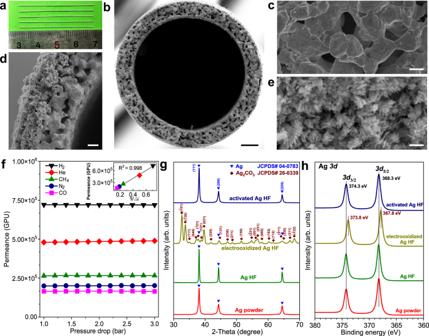Fig. 2: Structural and compositional characterization. aOptical image of the as-fabricated Ag HF tubes. SEM images ofb,d, cross sections andc,e, outer surfaces ofb,c, Ag HF andd,e, activated Ag HF. Scale bars inb,c,dandeare 50 µm, 5 µm, 10 µm and 500 nm, respectively.fGas permeances of activated Ag HF. GPU denotes gas permeation unit. Inset: the permeances (at 1.0 bar) are proportional to the inverse square root of gas molecular weight.gXRD patterns, andh, XPS spectra of Ag HF and activated Ag HF. {Ag}/{AgCl}\right)+0.197V+0.0591V\times {pH}+0.85i{R}_{s}\) , where E (vs. Ag/AgCl) is the applied potential, pH is the pondus hydrogenii value of the electrolyte solutions with different concentrations (Supplementary Table 2 ), i is the current density at each applied potential, and R s is the solution resistance obtained by EIS measurements (Supplementary Table 2 ), and 85% iR compensation was applied to correct the potential manually. All applied potentials in the main text and Supplementary Information referred to the RHE unless otherwise stated. CO 2 electroreduction tests The potentiostatic electroreductions of CO 2 over all electrodes were performed at ambient temperature and pressure on the Biologic VMP3 potentiostat using the gas-tight electrolysis cell. 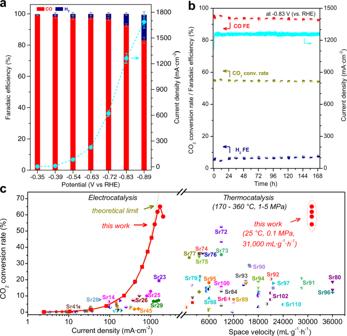Fig. 3: Performance of activated Ag HF. aCO and H2faradaic efficiencies, and total current densities in the potential range of −0.35 to −0.89 V. Error bars inawere obtained from the average of six individual tests.bLong-term performance at −0.83 V.cCO2conversion rates with a space velocity of 31,000 mL · gcat−1· h−1at different current densities, and their overall comparison with other electrocatalytic and thermocatalytic CO2conversions. All comparison data points incare from the references summarized in Supplementary TableS1, and the key data points are referred to the corresponding Supplementary references Srx, where x represents the reference number inSupplementary Information. CO2-saturated 1.5 M KHCO3as the electrolyte solution, and the CO2flow rate of 60 mL · min−1. The cathodic and anodic compartments were separated by a Nafion 117 membrane, and the electrolysis cell was equipped with a KCl-saturated Ag/AgCl reference electrode in the cathodic compartment and a platinum mesh counter electrode in the anodic compartment. 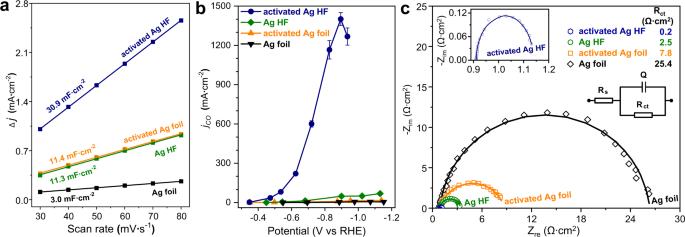Fig. 4: Electrochemical characterization. aPlot ofΔj(the difference of cathodic and anodic current densities,jc–ja) against the scan rates from cyclic voltammetry curves (Supplementary Fig.16),bCO partial current density comparison, and error bars were obtained from the average of six individual tests.cEIS Nyquist plots of activated Ag HF, Ag HF, activated Ag foil and Ag foil. The inset incshows the equivalent circuit. More details can be found in Supplementary CO 2 Electroreduction and Product Quantifications section as well as Supplementary Fig. 14 . Isotopic trace The isotope-labelling experiments were conducted under the same electrolysis reaction conditions that used C 18 O 2 and D 2 O as feedstocks. The feedstocks were supplied into the cathodic and anodic compartments of the electrolysis cell according to the following four situations: ( I ) nonisotope-labeled CO 2 was fed to the cathodic compartment, and nonisotope-labeled H 2 O was used as the solvent in the anodic compartment; ( II ) nonisotope-labeled CO 2 was fed to the cathodic compartment, and D-labeled D 2 O was used as the solvent in the anodic compartment; ( III ) 18 O-labeled C 18 O 2 was fed to the cathodic compartment, and nonisotope-labeled H 2 O was used as the solvent in the anodic compartment; ( IV ) 18 O-labeled C 18 O 2 was fed to the cathodic compartment, and D-labeled D 2 O was used as the solvent in the anodic compartment. The gas-phase exhausts from the cathodic compartment were first vented into 10 M NaOH solution to absorb unreacted CO 2 , and then the residual gases were detected by mass spectrometry (MS, GSD320-OmniStar, Pfeiffer Vacuum Corp., Germany). The offline catholyte sampled after 30-min electrolysis was placed into a water bath of 80 °C and then introduced into the mass spectrometer by a CO 2 flow of 10 mL ∙ min −1 . The MS data were analyzed and identified using QUADERA Version 4.60 software. Time-resolved operando Raman spectroscopy Time-resolved operando Raman measurements were carried out on a Raman spectrometer (i-Raman Pro BWS475-532H, B&W Tek Corp.) using a 532 nm excitation laser with a laser power of 25 mW. The Raman shift was calibrated to 520 cm −1 using a Si wafer. Activated Ag HF and activated Ag foil were used as the working electrodes in the electrolysis cell for the operando Raman measurements, respectively. The electrolyte solution was CO 2 -saturated 1.5 M KHCO 3 and the CO 2 flow rate was kept at 60 mL∙min −1 for all Raman measurements. In order to decrease the disturbance of bubbles, the focus points of all Raman tests were generally close to the bottom region of the hollow fiber electrodes, where the bubbles were relatively sparse (Supplementary Fig. 11d ). Raman spectra at the stable states of CO 2 electroreduction over a wider range of 300 to 2000 cm −1 were also obtained for the purpose of identifying the peaks from adsorbed bicarbonate ions or other possible species (Supplementary Fig. 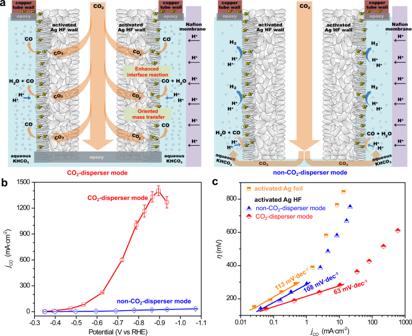Fig. 5: CO2dispersion effect studies. aSchematic illustrations showing the processes of CO2electroreduction over activated Ag HF with the CO2-disperser mode and the non-CO2-disperser mode, respectively, andb, their CO partial current densities. Error bars inbwere obtained from the average of six individual tests.cTafel slopes of activated Ag foil and activated Ag HF with different dispersion modes. 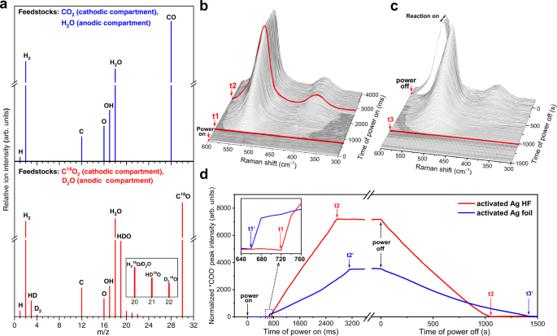Fig. 6: Isotopic trace and time-resolved operando Raman results. aMass spectrometric detections of the cathodic products over activated Ag HF using unlabeled feedstocks (upper) and isotopically labeled C18O2and D2O feedstocks (lower), respectively.b,cTime-resolved operando Raman spectra showing the formation, evolution and dissipation of intermediates over activated Ag HF.dComparison of the normalized *COO−peak intensities of activated Ag HF and activated Ag foil during the power-on and power-off stages. 20 ). Operando Raman spectra were recorded continuously within a range of 300 to 600 cm −1 without any time intervals (Supplementary Fig. 21 ), and in the meantime the potentials of CO 2 electroreduction were fixed at −0.83 and −0.69 V for activated Ag HF and activated Ag foil, respectively, which corresponded to their favorable electrocatalytic performance, i.e., ~1.26 A · cm −2 for activated Ag HF and 12 mA · cm −2 for activated Ag foil. Each Raman curve was obtained using a commercially available data-processing program (BWSpec 4.11 software), which was further subjected to smoothing treatment using commercial Origin 9.2 software before assembly of the operando Raman spectra. In addition, frequent power-on and power-off switching was applied during CO 2 electroreduction, which was monitored by Raman spectra in a range of 300 to 600 cm −1 to confirm the reproducibility of the Stark effect in our tests (Supplementary Fig. 22 ).